A single-cell transcriptomic landscape of primate arterial aging 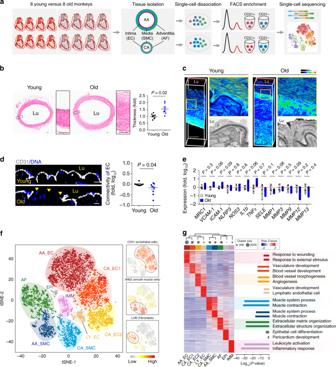Fig. 1: Diversity of cell types identified by scRNA-seq analysis. aMethod flowchart. Aortic artery (AA), coronary artery (CA), endothelial cell (EC), smooth muscle cell (SMC) and adventitial fibroblast (AF). b, Hematoxylin/eosin staining (left) and the calculated wall thickness (right) in vessel tissues from young and old monkeys. Rectangle, enlarged area. Scale bar, 100 μm.cLarge-scale three-dimensional reconstruction of a rectangular piece of vascular wall using automatic collector of ultrathin sections scanning electron microscopy (AutoCUTS-SEM). Left, volume electron microscopy. Upper right corner, enlarged area within the yellow rectangle. Lower right corner, representative section from the position of the red line before coloring with Imaris9.2.1 (color-key). See also Supplementary Fig.1g. Scale bar, 100 or 10 μm.dLeft, immunofluorescence staining for CD31 in young and old monkey vessels in the vicinity of aortic arch. Right, quantification of the connectivity between ECs. Yellow arrowheads indicate points of disconnection between ECs in old monkeys. Scale bar, 25 μm.eBulk qPCR of proatherosclerotic and atherosclerotic genes in both young and old monkey vessels.fThe position of the major cell classes in a t-SNE diagram (Left), as annotated using marker expression (Right). AA_EC, ECs mainly from the aortic arch; CA_EC1, CA_EC2, and LY_EC, three subgroups of ECs mainly from the coronary vasculature; AA_SMC, smooth muscle cells mainly from aortic arch; CA_SMC, smooth muscle cells mainly from coronary arteries; AF adventitial fibroblasts, IMM immune cells, EPI epicardial cells. Right, expression of known markers (gray, no expression; deep red, relatively high expression).gCell type expression signatures. GO terms are shown to the right. Lu lumen. Data are presented as mean ± SEM;n= 8 monkeys (b,d,e).Pvalues were determined by two-tailed Student’sttest (b,d) or one-way ANOVA followed by Holm-Sida’s multiple comparisons test (e). Our understanding of how aging affects the cellular and molecular components of the vasculature and contributes to cardiovascular diseases is still limited. Here we report a single-cell transcriptomic survey of aortas and coronary arteries in young and old cynomolgus monkeys. Our data define the molecular signatures of specialized arteries and identify eight markers discriminating aortic and coronary vasculatures. Gene network analyses characterize transcriptional landmarks that regulate vascular senility and position FOXO3A , a longevity-associated transcription factor, as a master regulator gene that is downregulated in six subtypes of monkey vascular cells during aging. Targeted inactivation of FOXO3A in human vascular endothelial cells recapitulates the major phenotypic defects observed in aged monkey arteries, verifying FOXO3A loss as a key driver for arterial endothelial aging. Our study provides a critical resource for understanding the principles underlying primate arterial aging and contributes important clues to future treatment of age-associated vascular disorders. Cardiovascular disorders (i.e., atherosclerosis) are leading causes of morbidity and death worldwide. Aging is a major risk factor for cardiovascular disease [1] . Age-associated changes in arterial properties, such as endothelial dysfunction and structural alterations, are considered to be initial events in the development of atherosclerosis [2] . The aortic and coronary arteries are two of the most lesion-susceptible regions in the human vasculature with age [3] , [4] , [5] . However, it is ethically and technically difficult to obtain and isolate aortic and coronary arteries from young and old individuals who have no manifestation of cardiovascular malfunction. Instead, monkeys are similar to humans in terms of their genetic, anatomical and physiological features, and their sensitivity to aging-related diseases [6] , [7] , thus representing an ideal model for studying vascular aging and related diseases. Forkhead box O3A (FOXO3A) is an evolutionarily conserved transcription factor (TF) that influences lifespan in model organisms [8] . FOXO3A genotype correlates with longevity traits in Asian and European populations [8] . Certain single-nucleotide polymorphisms of human FOXO3A are also associated with a lower prevalence of cardiovascular disease in long-lived humans [9] . Although considerable advances have been made in the molecular characterization of FOXO3A [8] , whether FOXO3A plays a geroprotective role in primate (including human) vasculature remains largely elusive. The development of therapeutic strategies to delay vascular aging and treat atherosclerosis requires accurate analyses of the cellular components and molecular properties of the aged human vessels. Single-cell sequencing of senile vasculature allows mapping of the diverse cellular landscapes and identification of cell type specific regulatory changes during aging [6] , [10] , [11] . Here, we obtain single-cell transcriptomic atlas of the atherosclerosis-prone aortic arch and coronary artery in young and aged nonhuman primates, cynomolgus monkeys. Based on this dataset, we identify unique molecular signatures illustrating aorta- and coronary artery-specific cell diversity. More importantly, we reveal cell type specific changes in molecular programs of aged primate vasculature. Besides, we identify FOXO3A as a central protective factor safeguarding primate vascular homeostasis. Targeted inactivation of FOXO3A in human arterial vascular endothelial cells (ECs), which results in the disruption of cellular homeostasis, recapitulates the major phenotypic defects observed in aged monkey arteries. Thus, our work provides a comprehensive understanding of aortic and coronary vasculature aging at single-cell level, which paves the way for new therapies against human cardiovascular diseases. scRNA-seq analysis of young and old monkey aortic and coronary arteries To study the subpopulation structure and molecular characteristics of the aged monkey vasculature, we performed single-cell RNA sequencing (scRNA-seq) on lesion-prone aortas and coronary arteries sampled from eight young (age, 4–6 years) and eight old (age, 18–21 years) cynomolgus monkeys (Fig. 1a , Supplementary Fig. 1a , and Supplementary Data 1 ). All monkeys were identified as healthy individuals without significant features of atherosclerosis (Supplementary Fig. 1b–d ). Morphologically, senile aortas exhibited characteristics of vascular aging, including increased wall thickness, fibrous cap formation, arterial calcification and fragmentation of the elastic lamina, determined by histological analysis and large-scale three-dimensional reconstruction using an automatic collector of ultrathin sections scanning electron microscope (AutoCUTS-SEM) (Fig. 1b, c , Supplementary Fig. 1e–g and Supplementary Movies 1 – 4 ) [12] . Moreover, denuded endothelial surfaces appeared in the aged intima (Fig. 1d ) [2] . Despite these morphological disturbances in aged vessels, we did not observe any significant upregulation of atherosclerogenic genes by analyzing transcripts in bulk vascular tissues (Fig. 1e ) [13] , highlighting the importance of decoding age-associated vascular transcriptomics at the single-cell resolution [14] . Fig. 1: Diversity of cell types identified by scRNA-seq analysis. a Method flowchart. Aortic artery (AA), coronary artery (CA), endothelial cell (EC), smooth muscle cell (SMC) and adventitial fibroblast (AF) . b , Hematoxylin/eosin staining (left) and the calculated wall thickness (right) in vessel tissues from young and old monkeys. Rectangle, enlarged area. Scale bar, 100 μm. c Large-scale three-dimensional reconstruction of a rectangular piece of vascular wall using automatic collector of ultrathin sections scanning electron microscopy (AutoCUTS-SEM). Left, volume electron microscopy. 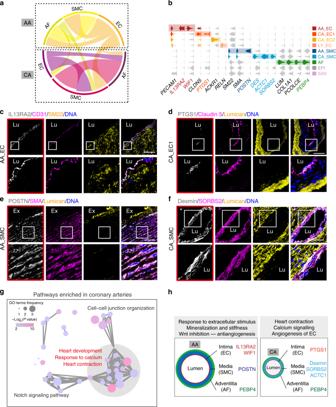Fig. 2: Survey of scRNA expression of cells from the aortic artery and the coronary artery. aThe transcriptomic profiling of aortic EC, SMC, and AF were compared with that of coronary arterial EC, SMC, and AF, respectively. Circos plot showing these site-specific genes were mainly shared by various cell populations from the same vascular bed. Lines, shared genes.bViolin plots of representative cell type specific markers. See Fig.1for cell-type abbreviations.cImmunofluorescence staining shows IL13RA2 (marker for AA_EC) expression in endothelial cells from the aortic artery. See also Supplementary Fig.4b.dImmunofluorescence staining shows PTGS1 (marker for CA_EC1) expression in endothelial cells from the coronary artery. See also Supplementary Fig.4c.eImmunofluorescence staining shows POSTN (marker for AA_SMC) expression in smooth muscle cells from the aortic artery. See also Supplementary Fig.4d.fImmunofluorescence staining shows that Desmin and SORBS2 are markers for CA_SMC and both are expressed in smooth muscle cells from coronary arteries. See also Supplementary Fig.5band c. Scale bars (c–f), 50 μm. White squares (c–f) correspond to enlarged areas shown in the lower images. (c–f) Lu lumen; Ex extravascular space.gNetworks of region-specific GO terms summarized by REVIGO. Differentially expressed genes (DEGs) between similar cell types (AA_EC vs. CA_EC1, AA_SMC vs. CA_SMC, AA_AF vs. CA_AF), were used to perform a GO analysis. Node colors indicate the –log2(pvalue);pvalues were corrected by the Benjamini-Hochberg algorithm; node size indicates the frequency with which the individual GO terms appeared. GO terms that are highly similar are linked by edges in the graph.hSchematic illustration of vascular organotypicity with region-specific markers and pathways. Upper right corner, enlarged area within the yellow rectangle. Lower right corner, representative section from the position of the red line before coloring with Imaris9.2.1 (color-key). See also Supplementary Fig. 1 g. Scale bar, 100 or 10 μm. d Left, immunofluorescence staining for CD31 in young and old monkey vessels in the vicinity of aortic arch. Right, quantification of the connectivity between ECs. Yellow arrowheads indicate points of disconnection between ECs in old monkeys. Scale bar, 25 μm. e Bulk qPCR of proatherosclerotic and atherosclerotic genes in both young and old monkey vessels. f The position of the major cell classes in a t-SNE diagram (Left), as annotated using marker expression (Right). AA_EC, ECs mainly from the aortic arch; CA_EC1, CA_EC2, and LY_EC, three subgroups of ECs mainly from the coronary vasculature; AA_SMC, smooth muscle cells mainly from aortic arch; CA_SMC, smooth muscle cells mainly from coronary arteries; AF adventitial fibroblasts, IMM immune cells, EPI epicardial cells. Right, expression of known markers (gray, no expression; deep red, relatively high expression). g Cell type expression signatures. GO terms are shown to the right. Lu lumen. Data are presented as mean ± SEM; n = 8 monkeys ( b , d , e ). P values were determined by two-tailed Student’s t test ( b , d ) or one-way ANOVA followed by Holm-Sida’s multiple comparisons test ( e ). Full size image By fluorescence-activated cell sorting (FACS)-mediated separation of CD31-positive ECs (CD31 + , also known as PECAM1) and CD31-negative (CD31 − ) cells (Fig. 1a ) and subsequent combination of all the information of cells from the aortic and coronary arteries, we obtained 7,989 high-quality vascular wall cells (3658 cells from young individuals and 4331 cells from old individuals) and detected an average number of 3112 genes per cell (Supplementary Data 1 ), with the housekeeping gene ACTB comparably expressed across samples (Supplementary Fig. 2a, b ) [15] . The cells from vascular walls were grouped into nine clusters, consistent with the enrichment strategy and anatomical regions, and were able to be mapped to the tunica intima , media , and adventitia of arterial vessels (Fig. 1f and g and Supplementary Fig. 2c–e ). Annotation of ECs, smooth muscle cells (SMCs), and adventitial fibroblasts (AFs) from different tunica layers were guided by the expression status of canonical cell type specific markers, as exemplified in Fig. 1f . In addition to endothelial and mural cells, we obtained clusters corresponding to lymphatic EC-like cells (LY-EC, RELN + and FLT4 + ), epicardial cells (EPI, KRT19 + and MSLN + ), and immune cells (IMM, CD68 + and CD83 + ) (Supplementary Fig. 2 f) [11] . Site-specific gene expression signatures of aortic and coronary arteries We next compared the single-cell transcriptomes from aortic and coronary arteries. Differentially expressed genes (DEGs) were separately identified between aortic and coronary ECs, between aortic and coronary SMCs, and between aortic and coronary fibroblasts. Circos plot showed that aortic and coronary cells exhibited site-specific gene expression signatures (Supplementary Figs. 3 – 5 ), which were mainly shared by various cell populations from the same vascular bed (Fig. 2a ). As verified by immunofluorescence analysis, a panel of location-specific genes were differentially expressed between cells from aortic and coronary arteries (Fig. 2b–f , Supplementary Fig. 2f , and Supplementary Figs. 4 , 5 ). We observed that SOST , a Wnt antagonist [16] , was highly expressed within all three layers of aortic arteries (Supplementary Fig. 4a ), consistent with a previous report that SOST expression is restricted to the great arteries [16] . IL13RA2 and WIF1 were identified as characteristic markers of aortic ECs (Fig. 2b, c , and Supplementary Fig. 4b ), whereas PTGS1 was uniquely expressed in coronary ECs (Fig. 2b , d, and Supplementary Fig. 4c ). Of note, WIF1 is also a Wnt antagonist inhibiting EC proliferation and angiogenesis, while PTGS1 promotes angiogenesis in ECs [17] , [18] . As for the middle coat ( tunica media ), the aortic SMCs expressed a higher level of POSTN (Fig. 2b , e, and Supplementary Fig. 4d ), an extracellular matrix (ECM) protein highly expressed in the periosteum and related to bone density, than did coronary SMCs. Aortic arteries also expressed OMD (also called osteomodulin) (Supplementary Fig. 4a ), which is a component of the ECM and is thus important for bone mineralization [19] . In contrast, coronary SMCs preferentially expressed DES , ACTC1 , and SORBS2 , which are also highly expressed in cardiac muscles [20] . Thus, the expression of these region-specific markers suggests that aortic arteries may have a lower angiogenesis ability and higher stiffness than the coronary arteries. In line with the function of these marker genes, Gene Ontology (GO) and KEGG analysis showed that aortic cells were primarily associated with the KEGG term “response to extracellular stimuli” (Supplementary Fig. 3 ); in contrast, vascular cells from the coronary arteries exhibited a predominance of pathways that regulate heart contraction and calcium signaling (Fig. 2g and Supplementary Fig. 3 ). In addition, we identified PEBP4 as a marker for AFs (Supplementary Fig. 5d ). Compared with the single-cell transcriptomic data of the rat aorta [11] , we found that IL13RA2 and WIF1 were specifically highly expressed in the ECs from the monkey aorta (Fig. 2b and Supplementary Fig. 4e ), implying the possible acquisition of primate-specific molecular markers of vessel identity during evolution. Altogether, these results defined the molecular signatures and functional heterogeneity of various arteries, suggesting that the molecular landscape underlining vascular organotypicity is programmed to adapt to region-specific arterial functions (Fig. 2h ). Fig. 2: Survey of scRNA expression of cells from the aortic artery and the coronary artery. a The transcriptomic profiling of aortic EC, SMC, and AF were compared with that of coronary arterial EC, SMC, and AF, respectively. Circos plot showing these site-specific genes were mainly shared by various cell populations from the same vascular bed. Lines, shared genes. b Violin plots of representative cell type specific markers. See Fig. 1 for cell-type abbreviations. c Immunofluorescence staining shows IL13RA2 (marker for AA_EC) expression in endothelial cells from the aortic artery. See also Supplementary Fig. 4b . d Immunofluorescence staining shows PTGS1 (marker for CA_EC1) expression in endothelial cells from the coronary artery. See also Supplementary Fig. 4c . e Immunofluorescence staining shows POSTN (marker for AA_SMC) expression in smooth muscle cells from the aortic artery. See also Supplementary Fig. 4d . 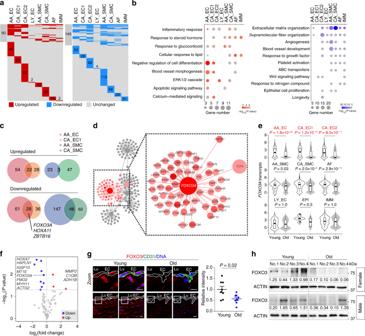Fig. 3: Gene regulatory network uncovers FOXO3A at the hub of aging regulation. aHeatmap showing the differentially expressed genes (O/Y DEGs, Bonferroni-correctedpvalue ≤ 0.05 and log2[fold change] ≥ 0.5) for each cell type from young and old monkeys.Pvalues were determined by two-sided Wilcoxon rank sum tests. Rows represent genes and columns are cell types. Red, upregulated genes; blue, downregulated genes; gray, genes not differentially expressed. The number of O/Y DEGs in at least two cell populations is shown in the gray rectangles; the number of O/Y DEGs uniquely differentially expressed in each cell type is shown in the colored rectangles. See Fig.1for cell-type abbreviations.bGO analysis of differentially expressed genes. Red, upregulated pathways; blue, downregulated pathways.cVenn diagrams of upregulated and downregulated genes shared in AA_EC/SMC and CA_EC1/SMC of old monkeys.dNetwork visualization of potential transcriptional regulation in the vessels. Node size is positively correlated with the number of directed edges. Nodes and edges that directly bind to the node ofFOXO3Aare highlighted in red; others are gray. Red is positively correlated with the number of motif-binding sites (darker red reflects more motifs). Dashed square, enlarged area.eViolin plots with box plots inside showingFOXO3Aexpression across cell types.fVolcano plot of O/Y DEGs (pvalue ≤ 0.05, two-sided Student’sttest) verified by qPCR. Blue dots, downregulated genes; red dots, upregulated genes.gLeft, immunofluorescence staining for FOXO3A and CD31 in the aortic artery. Right, quantification of immunofluorescence intensity in young and old vessel samples. Lu lumen, EC endothelial cells. Scale bar, 10 μm. Data are presented the means ± SEM;n= 8 monkeys;pvalues were determined by two-sided Student’sttest.hWestern blotting and band intensity quantification of FOXO3 protein levels in young and old vessel samples. 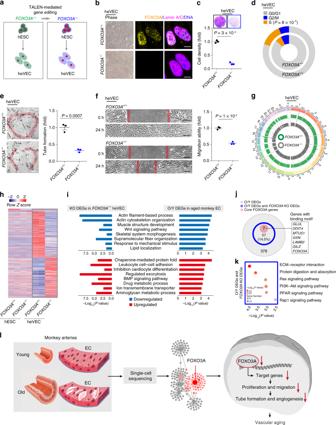Fig. 4: FOXO3A−/−ECs exhibited impaired cell proliferation and migration. aSchematic showing the method used to generateFOXO3A+/+andFOXO3A−/−heVECs.bRepresentative bright-field and immunostaining for FOXO3A inFOXO3A+/+andFOXO3A−/−heVECs. Scale bar, 50 or 5 μm.cUpper, clonal expansion analysis ofFOXO3A+/+andFOXO3A−/−heVECs. Bottom, areas positive for crystal violet staining were quantified by ImageJ.n= 3 independent experiments. Scale bar, 100 µm.dThe percentage of heVECs at each cell-cycle stage.n= 3 independent experiments.eIn vitro angiogenesis is assessed by the formation of capillary-like tubes fromFOXO3A+/+andFOXO3A−/−heVECs. The red circle represents an intact tube.n= 4 independent experiments. Scale bar, 100 μm.fLeft, representative wound scratch assay for detecting changes inFOXO3A−/−heVECs migration compared with wild-type heVECs migration. Red lines represent scar boundaries.n= 3 independent experiments. Scale bar, 100 μm. Right, quantification of wound scratch assay results.gWhole-genome sequencing analysis of copy number variation (CNV) inFOXO3A+/+andFOXO3A−/−heVECs.hHeatmap showing all differentially expressed genes inFOXO3A+/+andFOXO3A−/−hESCs and heVECs.iTop eight GO terms shared by O/Y DEGs andFOXO3A+/+/FOXO3A−/−DEGs.jA diagram showing seven core FOXO3A-regulated genes, as defined by common genes between O/Y DEGs of aged monkey ECs,FOXO3AKO DEGs inFOXO3A+/+andFOXO3A−/−heVECs, and FOXO3A target genes predicted by SCENIC in aged monkeys.kKEGG pathway of 64 common genes overlapped between O/Y DEGs of aged monkey ECs andFOXO3AKO DEGs of heVECs.lA working model for FOXO3A in the homeostatic regulation of aged primate vessels. Data are presented as mean ± SEM;pvalues were determined by two-sided Student’sttest (c–f) or corrected by the Benjamini–Hochberg algorithm (i,k). f Immunofluorescence staining shows that Desmin and SORBS2 are markers for CA_SMC and both are expressed in smooth muscle cells from coronary arteries. See also Supplementary Fig. 5b and c. Scale bars ( c – f ), 50 μm. White squares ( c – f ) correspond to enlarged areas shown in the lower images. ( c – f ) Lu lumen; Ex extravascular space. g Networks of region-specific GO terms summarized by REVIGO. Differentially expressed genes (DEGs) between similar cell types (AA_EC vs. CA_EC1, AA_SMC vs. CA_SMC, AA_AF vs. CA_AF), were used to perform a GO analysis. Node colors indicate the –log 2 ( p value); p values were corrected by the Benjamini-Hochberg algorithm; node size indicates the frequency with which the individual GO terms appeared. GO terms that are highly similar are linked by edges in the graph. h Schematic illustration of vascular organotypicity with region-specific markers and pathways. Full size image Cell type specific transcriptional changes of senile primate arteries Next, we investigated age-related changes based on single-cell datasets. We observed minimal age-related biases in cell-type clustering between cells from young and old monkeys (Supplementary Fig. 2d–e and Supplementary Data 1 ). We then compared cell-intrinsic gene expression programs of the same cell types between young and old monkeys and identified 515 downregulated and 259 upregulated genes (log 2 [fold change] ≥ 0.5 and adjusted p value ≤ 0.05, referred to as old/young differentially expressed genes, O/Y DEGs) that were differentially expressed in at least one type of vascular cells (Fig. 3a and Supplementary Fig. 6a ). The core pathways annotated for upregulated O/Y DEGs that were shared by diverse vascular cell types involved several atherosclerosis-related pathways, such as calcium signaling, response to lipids, and inflammatory response (Fig. 3b ) [21] . By comparison, annotated pathways for downregulated O/Y DEGs that were shared by disparate vascular cell types included ECM organization, angiogenesis, and Wnt signaling pathway (Fig. 3b ). These observations were consistent with the compromised endothelial barriers, increased arterial calcification, and fragmentation of the elastic lamina that we observed in aged monkey arteries (Fig. 1b–d and Supplementary Fig. 1e, f ). However, only ~20% of O/Y DEGs were shared by at least two cell populations (Fig. 3a and c ); the majority of O/Y DEGs were cell type- and anatomical origin-specific (Fig. 3a and c ). To identify the differential molecular programs underlying aortic and coronary artery aging, we compared the biological functions of cell type specific O/Y DEGs between aortic arches and coronary arteries via GO analysis and found that aged aortic arches were more sensitive to blood coagulation and various external stimuli, while coronary arteries were more susceptible to infection and leukocyte activation (Supplementary Fig. 7a ). Thus, vascular cells from disparate anatomical locations exhibited both common and unique features related to erosive vascular changes during aging. Given that an increase in transcriptional instability has been regarded as one of the features of mammalian aging [22] , we investigated transcriptional noise during monkey vascular aging. As expected, age-dependent transcriptional noise accumulated in the intima and adventitia of both aortic and coronary arteries, particularly in the ECs (Supplementary Fig. 7b ). GO analysis of genes with high transcriptional variability during aging revealed that cell-to-cell variation increased in response to lipid stimulation and inflammation (Supplementary Fig. 7c ). Fig. 3: Gene regulatory network uncovers FOXO3A at the hub of aging regulation. a Heatmap showing the differentially expressed genes (O/Y DEGs, Bonferroni-corrected p value ≤ 0.05 and log 2 [fold change] ≥ 0.5) for each cell type from young and old monkeys. P values were determined by two-sided Wilcoxon rank sum tests. Rows represent genes and columns are cell types. Red, upregulated genes; blue, downregulated genes; gray, genes not differentially expressed. The number of O/Y DEGs in at least two cell populations is shown in the gray rectangles; the number of O/Y DEGs uniquely differentially expressed in each cell type is shown in the colored rectangles. See Fig. 1 for cell-type abbreviations. b GO analysis of differentially expressed genes. Red, upregulated pathways; blue, downregulated pathways. c Venn diagrams of upregulated and downregulated genes shared in AA_EC/SMC and CA_EC1/SMC of old monkeys. d Network visualization of potential transcriptional regulation in the vessels. Node size is positively correlated with the number of directed edges. Nodes and edges that directly bind to the node of FOXO3A are highlighted in red; others are gray. Red is positively correlated with the number of motif-binding sites (darker red reflects more motifs). Dashed square, enlarged area. e Violin plots with box plots inside showing FOXO3A expression across cell types. f Volcano plot of O/Y DEGs ( p value ≤ 0.05, two-sided Student’s t test) verified by qPCR. Blue dots, downregulated genes; red dots, upregulated genes. g Left, immunofluorescence staining for FOXO3A and CD31 in the aortic artery. Right, quantification of immunofluorescence intensity in young and old vessel samples. Lu lumen, EC endothelial cells. Scale bar, 10 μm. Data are presented the means ± SEM; n = 8 monkeys; p values were determined by two-sided Student’s t test. h Western blotting and band intensity quantification of FOXO3 protein levels in young and old vessel samples. Full size image To identify the master regulators (MRs) related to vascular aging, we constructed gene regulatory networks of transcription factors and their target genes using the SCENIC workflow and identified six transcription factors ( FOXO3A, TCF3, GLISI, NFIX, TGIF1, and RBPJ ) with recognition motifs that were significantly enriched in the cis -regulatory elements of co-expressed gene sets (Fig. 3d , Supplementary Data 2 ) [23] . As shown in the network topology, FOXO3A acted as a top regulatory hub with the highest number of target genes involved in primate arterial aging (Fig. 3d , Supplementary Data 2 ). We also used ARACNe and VIPER algorithms to generate interactomes of all O/Y DEGs (see also “Method” section). The interactomes also pointed to FOXO3A as a top MR (Supplementary Fig. 8a and b ) [24] . GO analysis of O/Y DEGs with FOXO3A binding motifs in the transcriptional network identified three characteristics: (1) regulation of the immune system (e.g., COLEC10 , ZBTB16 , and TCF3 ), (2) positive regulation of cell proliferation and migration (e.g., MYC and THBS4 ) and (3) response to insulin and lipid (e.g., PIK3R1, SORBS1 , and TXNIP ) (Supplementary Fig. 8c ). These characteristics were also core features compromised in senile vessels (Fig. 3b ). Furthermore, we compared O/Y DEGs, with cardiovascular disease-related genes database and aging/longevity-related genes from the GenAge database (Supplementary Fig. 8d–e ) [25] , [26] . These data further pinpointed FOXO3A , in addition to the known aging genes including Klotho , APOE , APOA1 , and SERPINE1 , as a candidate molecular culprit underlying vascular disease and aging [26] . Systematic analysis of differentially expressed transcripts between old and young monkey arteries further revealed 28 downregulated and 22 upregulated genes shared by disparate subtypes of ECs, among which only FOXO3A , HOXA11 , and ZBTB16 encoded transcription factors (Fig. 3c ). Analysis by scRNA-Seq further demonstrated that FOXO3A transcripts decreased in six vessel cell types, especially in ECs (log 2 [fold change] ≥ 0.5 and adjusted p value ≤ 0.05) (Fig. 3e ). Diminished FOXO3 transcript and protein levels in senile monkey arteries were verified by qPCR, Western blotting and immunofluorescence analyses (Fig. 3f–h , Supplementary Fig. 8f and Supplementary Data 3 ). Given that the longevity-associated single-nucleotide polymorphisms of FOXO3A have also been linked to the lower-than-average prevalence of cardiovascular disorders in centenarians [27] , we next focused on the potential role of FOXO3A in maintaining primate vasculature homeostasis. FOXO3A is a central protective factor in safeguarding vascular homeostasis To characterize how the loss of FOXO3A affects the function of vascular ECs, we first silenced FOXO3A expression using small interfering RNAs (siRNAs) in human aortic endothelial cells (HAECs) and human umbilical vein endothelial cells (HUVECs) (Supplementary Fig. 9a–d ). Consistent with previous findings [28] , the knockdown of FOXO3A enhanced tube formation ability of HUVECs (Supplementary Fig. 9f ). In contrast, FOXO3A deficiency disturbed self-renewal and tube-formation abilities of HAECs (Supplementary Fig. 9e–f ), implying that FOXO3A may be geroprotective in a vascular cell type specific manner. We further explored the molecular mechanism underlying the age-related downregulation of FOXO3A in primate arterial ECs. By employing bioinformatics tools linked to comprehensive knowledgebases including GeneCards suite databases and Gene Transcription Regulation Database (GTRD), we predicted a panel of potential transcriptional regulators of FOXO3A gene, including FOXA2, EP300, HOXA9, KAT7, MYC, NRF1, RelA, TEAD1/4, and ZBTB16 (Supplementary Fig. 10a ). The expression levels of these proteins in the aged aorta were assessed by western blotting (Supplementary Fig. 10b ). Among these predicted transcriptional regulators, FOXA2, a MR of embryogenesis and a potential TF active at early stages of endothelial specification [29] , was the most upregulated gene in aged monkey vessels relative to the young ones (Supplementary Fig. 10c ). As deregulation of the developmental program is increasingly being recognized as an underlying mechanism for cellular aging in various tissues [30] , [31] , we next investigated whether the upregulation of FOXA2 in primate arterial ECs contributed to the silence of FOXO3A and cellular malfunction. Overexpression of FOXA2 in HAECs resulted in a loss of FOXO3A and compromised cell proliferation (Supplementary Fig. 10d–g ), whereas siRNA-mediated knockdown of FOXA2 upregulated FOXO3A expression and stimulated cell proliferation (Supplementary Fig. 10h–k ). Chromatin immunoprecipitation (ChIP) and luciferase reporter assays further demonstrated that FOXA2 was able to bind to FOXO3A promoter and transrepressed FOXO3A transcription in HAECs (Supplementary Fig. 10l–n ). Altogether, these results suggest that enhanced transcriptional suppression of FOXO3A by FOXA2 may be responsible for the age-associated decay of primate arterial ECs. Notably, FOXO3B , an intron-less reverse-transcribed copy of the canonical FOXO3A gene, has recently been identified to exist only in the human genome [32] . To gain insight into the mechanism underlying how specific FOXO3A deletion mediates arterial endothelial dysfunction, we generated FOXO3A -knockout (KO) human ECs by specifically knocking out FOXO3A in human embryonic stem cells (hESCs) using the TALEN-facilitated homologous recombination technique (Fig. 4a and Supplementary Fig. 11a ). A 1.3-kb left homologous arm was designed in the intron of FOXO3A , making it essentially impossible to affect the sequence of FOXO3B by homologous recombination, as demonstrated by genomic PCR and Sanger sequencing (Supplementary Fig. 11a–c ). Consequently, the transcript of FOXO3A , rather than that of FOXO3B , was specifically abolished in FOXO3A -deficient hESCs ( FOXO3A −/− hESCs) (Supplementary Fig. 11d ) and the absence of FOXO3A protein in FOXO3A −/− hESCs was verified by western blotting (Supplementary Fig. 11e ). Moreover, FOXO3A -edited hESCs exhibited normal pluripotency and genomic integrity (Supplementary Fig. 11f–i ). Fig. 4: FOXO3A −/− ECs exhibited impaired cell proliferation and migration. a Schematic showing the method used to generate FOXO3A +/+ and FOXO3A −/− heVECs. b Representative bright-field and immunostaining for FOXO3A in FOXO3A +/+ and FOXO3A −/− heVECs. Scale bar, 50 or 5 μm. c Upper, clonal expansion analysis of FOXO3A +/+ and FOXO3A −/− heVECs. Bottom, areas positive for crystal violet staining were quantified by ImageJ. n = 3 independent experiments. Scale bar, 100 µm. d The percentage of heVECs at each cell-cycle stage. n = 3 independent experiments. e In vitro angiogenesis is assessed by the formation of capillary-like tubes from FOXO3A +/+ and FOXO3A −/− heVECs. The red circle represents an intact tube. n = 4 independent experiments. Scale bar, 100 μm. f Left, representative wound scratch assay for detecting changes in FOXO3A −/− heVECs migration compared with wild-type heVECs migration. Red lines represent scar boundaries. n = 3 independent experiments. Scale bar, 100 μm. Right, quantification of wound scratch assay results. g Whole-genome sequencing analysis of copy number variation (CNV) in FOXO3A +/+ and FOXO3A −/− heVECs. h Heatmap showing all differentially expressed genes in FOXO3A +/+ and FOXO3A −/− hESCs and heVECs. i Top eight GO terms shared by O/Y DEGs and FOXO3A +/+ / FOXO3A −/− DEGs. j A diagram showing seven core FOXO3A-regulated genes, as defined by common genes between O/Y DEGs of aged monkey ECs, FOXO3A KO DEGs in FOXO3A +/+ and FOXO3A −/− heVECs, and FOXO3A target genes predicted by SCENIC in aged monkeys. k KEGG pathway of 64 common genes overlapped between O/Y DEGs of aged monkey ECs and FOXO3A KO DEGs of heVECs. l A working model for FOXO3A in the homeostatic regulation of aged primate vessels. Data are presented as mean ± SEM; p values were determined by two-sided Student’s t test ( c – f ) or corrected by the Benjamini–Hochberg algorithm ( i , k ). Full size image We subsequently derived human vascular ECs from hESCs (hereafter referred as to heVECs) with an optimized directed differentiation protocol (Supplementary Fig. 12a ) [33] . Single-cell RNA-sequencing analysis via 10× Genomics demonstrated that the majority of heVECs were bona fide ECs that expressed high levels of EC signatures, CD31 , CLDN5 , and ERG1 , and were relatively homogenous at single-cell resolution (Supplementary Fig. 12b and c ) [34] . Like HAECs, heVECs expressed canonical arterial EC markers, such as NRP1 , NOTCH1 , and DLL4 (Supplementary Fig. 12d–f ) [34] , [35] . Transposase-accessible chromatin followed by sequencing (ATAC-seq) further identified that the chromatin-binding sites of ETS family transcription factors as the master regulators for the maintenance of aortic endothelial identity were highly accessible in heVECs [36] , resembling their HAEC counterparts (Supplementary Fig. 12g and h ). Functionally, heVECs possessed the ability to form capillary-like structures and produce nitric oxide (NO) as did HAECs (Supplementary Fig. 12i and j ). Lastly, both heVECs and primary HAECs exhibited similar phenotypic defects such as compromised proliferation and tube formation abilities upon FOXO3A ablation, which was not the case for HUVECs (Supplementary Fig. 9c–f ). Thus, we successfully obtained heVECs with arterial characteristics which partially phenocopied HAECs. We next differentiated both wild-type and FOXO3A −/− hESCs into heVECs (Fig. 4a, b and Supplementary Fig. 13a ). Flow cytometry analysis revealed that the differentiation efficiency of FOXO3A −/− hESCs to heVECs was comparable to that of wild-type hESCs (Supplementary Fig. 13a, b ). Phenotypically, FOXO3A -deficient heVECs exhibited decreased cell proliferation and tubular network formation abilities, diminished migration ability (Fig. 4b–f , Supplementary Fig. 13c and d ), and impaired DiI-labeled acetylated low-density lipoprotein (DiI-Ac-LDL) uptake (Supplementary Fig. 13e ). To further evaluate the effect of FOXO3A deficiency on heVECs in a physiologically relevant context, we evaluated the vasculogenesis activity of FOXO3A −/− heVECs using a well-established hindlimb ischemia murine model and showed that FOXO3A deficiency in heVECs compromised vascular regeneration and repairability in vivo (Supplementary Fig. 13 f) [33] . These results were consistent with the observed erosion of the endothelium in old monkey arteries along with age-related downregulation of FOXO3A (Fig. 1b–d , Supplementary Fig. 1e, f). To explore the molecular events downstream of FOXO3A that regulate heVEC homeostasis, we performed genomic and transcriptomic analyses of FOXO3A −/− heVECs. Both FOXO3A −/− and wild-type heVECs were genomically stable, as indicated by genome-wide copy number variation (CNV) analyses (Fig. 4g ). We further observed 1404 upregulated and 1617 downregulated genes (log 2 [fold change] ≥ 0.5, adjusted p value ≤ 0.05, referred as to KO DEGs, Supplementary Data 4 ) in FOXO3A −/− heVECs in comparison with wild-type heVECs (Fig. 4h and Supplementary Fig. 14a ). Notably, deficiency of FOXO3A in heVECs led to changes in molecular pathways resembling those observed in the vascular ECs from aged monkeys (Fig. 4i ), further supporting that FOXO3A downregulation underlies primate arterial endothelial malfunction. Next, we compared the O/Y DEGs of monkey ECs (old vs. young) with the FOXO3A KO DEGs of human heVECs ( FOXO3A −/− vs wild-type). Among the 378 DEGs in aged monkey ECs (compared with the young ones), 64 genes were also differentially regulated in FOXO3A −/− heVECs compared with their wild-type counterparts (Fig. 4j and Supplementary Fig. 14a, b). These genes were predominantly enriched in GO terms associated with the ECM-receptor interactions and the peroxisome proliferators-activated receptor (PPAR) signaling pathway, etc. (Fig. 4k ). Furthermore, 6 out of 64 genes, GLUL , DDIT4 , MTUS1 , GSN , GILZ , and LAMB2 , were putative FOXO3A target genes with classic FOXO3A-binding motif (Fig. 4j and Supplementary Fig. 14c–e ). Differential expression of these genes was confirmed in wild-type and FOXO3A −/− heVECs by qRT-PCR. By ChIP-qPCR assay, we further verified the enrichment of FOXO3A in the upstream of GLUL (glutamine synthetase) gene (Supplementary Fig. 14d ), whose deletion has recently been reported to impair vessel sprouting and suppress angiogenesis [37] . Altogether, our data suggest that FOXO3A plays a guardian role in maintaining primate vascular homeostasis and its downregulation with age may be a key driver contributing to vascular disorders (Fig. 4l ). In this study, we developed a single-cell transcriptomic atlas of the atherosclerosis-prone aortic arch and coronary vasculature based on high-quality vascular wall cells from young and aged monkeys. Highlights of this work are enumerated here: (1) Characterized various tissue pathologies associated with physiological primate vascular aging, including increased wall thickness, arterial calcification, fibrous cap formation, fragmentation of elastic lamina and denuded endothelial surface. (2) Unraveled aortic artery- and coronary artery-specific molecular signatures for each vascular cell type. (3) Systematically dissected the aging-associated transcriptional landmarks linked to each cell type of the primate aortic and coronary arteries. (4) Uncovered the increase of transcriptomic noise particularly in vascular ECs and fibroblasts during primate aging. (5) Revealed the downregulation of a longevity gene FOXO3A in six vascular subpopulations in old monkeys relative to their young counterparts. (6) Identified FOXO3A as a central protective factor in safeguarding primate vascular homeostasis. (7) Suggested a geroprotective role of FOXO3A in EC origin-specific manner. (8) Demonstrated the critical role of a developmental regulator FOXA2, in the dysregulation of FOXO3A and endothelial malfunction during primate vascular aging. (9) Indicated the synergistic downregulation of a panel of core FOXO3A target genes during primate vascular aging. The findings on the cell type specific molecular programs underlying primate vascular aging provide a valuable resource to the geroscience community on top of the previous single-cell characterization of early progenitor cells that build coronary arteries [38] , cell classes and zonation in brain vasculature [39] , and immune cell population in mouse atherosclerosis [40] . Importantly, we identified FOXO3A as a central protective factor in safeguarding primate vascular homeostasis. FOXO3A is ubiquitously expressed across the body with tissue-restricted and lineage-specific functions in promoting healthspan and longevity [33] , [41] . Our study broadens and deepens the knowledge of FOXO3A ’s function in vascular biology by showing that FOXO3A deficiency compromised the tube formation and self-renewal abilities of HAECs and heVECs and that FOXO3A knockdown promoted HUVEC angiogenesis, consistent with the previous report [28] . Despite that heVECs obtained by optimized differentiation protocols [33] may not fully phenocopy primary aortic ECs, they exhibited comparative expression levels of arterial marker genes as did HAECs. By comparison, as HUVECs were derived from immune-privileged fetal tissue [42] , they may differ from adult vascular endothelium such as HAECs. Our data suggest that ECs from different origins (e.g. adult vs. embryonic; arterial vs. venous) may respond differently to FOXO3A deficiency and one possible explanation is that FOXO3A may regulate different downstream target genes in a cell type-dependent manner [43] as multiple FOXO3A target genes were identified by meta-analysis of our in vivo and in vitro datasets. In summary, our work provides a comprehensive understanding of primate aortic and coronary vasculature aging at single-cell level and supports a key role of FOXO3A downregulation in driving vascular dysfunction, which paves the way for new therapies against human vascular diseases. Animals All Macaca fascicularis were of Southeast Asian origin, including eight young (4–6 years old) and eight old (18–21 years old) monkeys. Animal rooms were maintained at ∼ 25 °C. Room lighting was automatically controlled on a 12-h light, 12-h dark schedule. Monkeys were fed a semi-purified, nutritionally fortified diet supplemented with one apple per day. Before this experiment, none of the monkeys had any history of a clinical disorder, experimental use that would be expected to affect physiological aging or disease susceptibility. Ultrasound-based imaging methods and blood tests were used to exclude animals with significant cardiovascular disease. All animals were raised at Xieerxin Biology Resource, an accredited primate research center in Beijing. This study was performed following the ethical guidelines of the Institutional Animal Care and Use Committee of the Institute of Zoology, Chinese Academy of Sciences. Two certified veterinarians supervised all animal experiments. All animal experiments complied with all relevant ethical regulations, and detailed information about the animals in this study is included in Supplementary Fig. 1a . Tissue isolation and cell dissociation To ensure successful isolation, we only acquired samples from one monkey per day (the animals fasted overnight before surgery). The entire process required a total of 16 sequential days in total. Monkey hearts with aortic arteries were surgically isolated under the expertise of certified veterinarians. The tissues were rinsed in cold Krebs–Henseleit solution (Anhui Leagene Biotechnology). The left and right coronary arteries branch from the root of the aortic arteries and rise from the anterior and posterior aortic sinus, respectively. To isolate coronary arteries from the heart, we first determined the location of the aortic sinus, carefully removed the epicardial tissue, and selected the left coronary artery running between the pulmonary trunk and the left auricle and extended to the vessel in the atrioventricular groove. The right coronary artery was identified between the pulmonary trunk and the right auricle and followed to the vessels in the posterior interventricular groove. Three regions of the coronary arteries, the right coronary arteries and the interventricular and circumflex branches of the left coronary artery, were carefully isolated from the surface of the monkey heart. However, due to the very limited size of coronary arteries, it may be unavoidable to be contaminated by nearby tissues which theoretically were discriminated by single-cell sequencing and subsequent analyses. Both the aortic arches and the coronary arteries were individually isolated and sliced into small fragments. The aortic arches and the coronary arteries were first digested by collagenase I (Thermo, 17100017) for 10 min, followed by digestion with a mixture of collagenase I, dispase II (Thermo, 17105041), elastase (Sigma, E7885), and DNase I (Worthington, LS006333) for 45 min. Then, the cell suspension was treated with Accumax (Thermo, 00-4666-56) for another 5 min to dissociate the cell aggregates into single cells. To enrich for CD31 + CD45 − ECs, the cell suspension was incubated with anti-CD31, anti-VE-cadherin, and anti-CD45 for 30 min, and FACS was used to separate positive and negative cells. Flow cytometry detection of the cell surface antigens and cell sorting were performed on a BD FACS Aria II with the indicated antibodies. Large-scale three-dimensional vessel reconstruction A volume electron microscopy technique called “automatic collector of ultrathin sections scanning electron microscopy” (AutoCUTS-SEM) was performed according to the published methods [12] . The workflow includes an automated hardware system for high throughput serial section collection, a software package for automatic SEM imaging, and an image reconstruction program. About 1300 sections were collected for each sample. Electron microscopy Electron microscopy was performed at the Center for Biological Imaging of the Chinese Academy of Sciences using a FEI Tecnai T12 G2 transmission electron microscope [44] . Single-cell RNA-seq library preparation and sequencing Single-cell RNA-seq libraries were prepared by using a modified protocol based on the STRT-seq protocol [6] . Briefly, after tissue digestion, single cells were picked into 2 μL cell lysis buffer with a mouth pipette under microscope. Reverse transcription was performed with oligo dT primers composed of 8 nt cell-specific barcodes, 8 nt unique molecular identifiers (UMI) and 25 nt oligo dT. The second-strand cDNA was synthesized followed by 19 cycles of PCR amplification with the 3′ P2 primer and the IS primer. Then, 96 different barcoded single-cell PCR preamplified products were pooled together and purified by AMPure XP beads (Beckman). Forty nanograms of DNA was then used to process four cycles PCR with IS primer and biotin-modified index primer. Index-induced cDNA was sheared to ~300 bp fragments by Covaris S2. Fragmented DNA was then enriched by incubating with streptavidin C1 beads (Thermo Fisher) for 1 h. Finally, the libraries were constructed using a KAPA Hyper Pre Kit (KAPA Biosystems). All single-cell RNA-seq data were generated on an Illumina HiSeq4000 platform for 150-bp paired-end reads [6] . Single-cell 3′ Library and Gel Bead Kit V3 (10× Genomics, 1000075) and Chromium Single Cell B Chip Kit (10× Genomics, 1000074) were used for cultured cells capture and cDNA synthesis. The cell suspension was loaded onto the Chromium single-cell controller (10× Genomics) to generate single-cell gel beads in the emulsion according to the manufacturer’s recommendation. Then, single cells were suspended in PBS containing 0.04% BSA. About 4000 cells were added to each channel, and the target cell recovery rate was estimated to be 2000 cells. Captured cells were lysed and the released RNA was barcoded through reverse transcription in individual GEMs. Reverse transcription was performed using an S1000TM Touch Thermal Cycler (Bio-Rad), the GEMs were programmed at 53 °C for 45 min, followed 85 °C for 5 min, and hold at 4 °C. The cDNA was generated and amplified, and the quality was assessed by the Agilent 4200 (performed by CapitalBio, Beijing). Sequencing was performed on the Illumina NovaSeq6000 sequencer with a sequencing depth of at least 100,000 reads per cell and 150 bp (PE150) paired-end reads (performed by CapitalBio, Beijing). Processing raw data from scRNA-seq of modified STRT-seq First, Reads2 of each library was split into data of single cells based on the 8-bp cell barcode, and then, the barcode with UMI information was attached to Reads1 according to the corresponding Reads2. After the template switch oligo, polyA and adapter sequences were trimmed from Reads1, and quality was controlled by removing reads shorter than 37 bp or reads with too many undetermined nucleotides ( N > 10%). Subsequently, clean reads were aligned to the genome of Crab-eating macaque (Macaca_fascicularis_5.0 sourced from Ensemble) using TopHat [45] , and annotations of some known markers based on NCBI prediction were included because they were not complete in the Ensemble Release 91 annotation files. Uniquely mapped reads were counted by HTseq [46] , and reads with the same UMIs were merged as one count. To exclude low-quality cells, only data from cells with 1000–10,000 genes, UMI counts of >3000, a mapping ratio >10%, 1.0 × 10 4 to 3.0 × 10 6 aligned reads, and genes with more than one transcript count in at least three cells were retained for further analysis. Processing raw data from scRNA-seq of 10× Genomics First, FASTQ files were processed by the function “cellranger count” of software CellRanger (10× Genomics, Version 3.0.2) to generate feature counts of every single cell. The reference genome was the human genome GRCh38 (10× Genomics, Version 3.0.0.). The total cells we obtained were 5210, the mean reads per cell were 126,807, the median number of genes for each cell was 5224, and the mean ratio of mitochondria per cell is 0.12. To remove the cells with low quality, cells with gene number over 2000, and the ratio of mitochondria lower than 0.15 were maintained, and genes with at least one feature count in more than three cells were used for the following analysis. Cell clustering of scRNA-seq data The filtered gene expression data of counts were analyzed by the Seurat (Version 2.1) package [6] , [47] , [48] . Global scaling normalization was applied with the “NormalizeData” function via the “LogNormalize” method and a scale factor 100,000 for modified STRT-seq and 10,000 for 10× scRNA-seq respectively according to their number of transcriptional counts. Highly variable genes were identified by “FindVariableGenes” and used for principal component analysis. Significant principal components that were enriched with low p value (≤1E-5) genes were used for cell clustering. The resolution of “FindClusters” was set to 0.5 for modified STRT-seq and 0.1 for 10× scRNA-seq respectively because the resulting clusters were consistent with the mapping of known markers. Identification of differentially expressed genes (DEGs) and biomarkers DEGs from scRNA-seq were identified by “FindAllMarkers” or “FindMarkers” using the “Wilcox” test, which returned “p_val_adj” using the Bonferroni correction and the log-transformed fold change, “avg_logFC”. Biomarkers of different clusters were selected from DEGs with p_val_adj ≤ 0.05 and avg_logFC ≥ 0.5. GO analysis GO analysis of biological process enrichment was performed using Metascape [49] ( http://metascape.org ) and GO ( http://www.geneontology.org ) [50] , [51] . Because most lists of GO terms are large and redundant, REVIGO was applied to summarize redundant GO terms based on semantic similarity measures [52] . Nonredundant GO term sets were visualized by Cytoscape, in which GO terms were set as nodes and 3% of GO term pairwise similarities were set as edges. Gene set enrichment analysis (GSEA) GSEA ( http://www.broadinstitute.org/gsea/index.jsp ) was performed to identify genes from an a priori-defined set that are different between two given cell types or groups [53] . The expression file, consisting of the top 5000 variable genes that were selected after employing the Seurat “FindVariableGenes” function, was loaded as input, and gene sets such as KEGG [54] pathways and GO were collected from the Molecular Signatures Database (MSigDB) [53] , [55] . Detection of transcriptional noise We improved the Euclidean distance-based method developed by Enge et al. [22] with some modifications to explain age-dependent transcriptional noise. Only genes expressed (counts ≥ 1) in at least three cells of each cell type were used to measure transcriptional noise. The noise was calculated as biological variation over technical variation. First, the Euclidean distance between each cell and the mean expression vector of each cell type of per-monkey were measured and divided by the technical Euclidean distance of ERCC spike-in controls. The distance of each cell in the old and young groups was summarized by the “compare_means” and “ggboxplot” functions of the “ggpubr” R package. Highly variable genes were selected from genes with “dispersion_empirical” three times of “dispersion_fit” by function “dispersionTable” of the Monocle package. TF-motif analysis The TF motif was found by the GENIE3 [56] and RcisTarget [57] R packages of the SCENIC [23] workflow using default parameters ( http://scenic.aertslab.org ). TFs of hg19 were used as reference TFs and downloaded using RcisTarget. GENIE3 inferred gene regulatory networks from the gene expression matrix of 7989 cells and 715 aging-related differentially expressed gene counts of each cell type. RcisTarget identified enriched TF-binding motifs and predicted candidate target genes (regulons) based on the database containing motifs with genome-wide rankings. Networks of the TF module with motif information were visualized by Cytoscape [58] . MR analysis MRs were identified by the ARACNe [24] algorithm and the VIPER [59] algorithm. First, interactomes of TFs and target genes were inferred by ARACNe ( https://sourceforge.net/p/aracne-ap/wiki/Home/ ) from hg19 TFs downloaded by RacisTarget. The input was normalized data sets for 7989 cells and the top 200 aging-related DEGs of each cell type. After obtaining the regulation network, MR analysis was performed using default settings by the viper package, which exploits the same principle as the MARINA [60] algorithm. The gene expression signature was defined by comparing the gene expression between the old and young monkeys. TFs with false discovery rate and p value less than 0.05 were selected as candidate MRs. Construct cell trajectories of each cell type along the pseudotime The Monocle2 [61] , [62] (version 2.6.1) package was applied to construct single-cell trajectories of cells of each cell type from a young state to an old state. DEGs in old and young monkeys for each cell type were identified by the “FindMarkers” function of the Seurat packages were set as “ordering_genes”. The DDRTree algorithm was used for dimensionality reduction. Modules of DEGs that covaried along the pseudotime were demonstrated by “plot_pseudotime_heatmap”. Identify regulators of FOXO3A gene To find the regulatory elements for the FOXO3 gene, we searched in the GeneCards database ( https://www.genecards.org/cgi-bin/carddisp.pl?gene=FOXO3 ) and selected TFs from “Transcription Factor Binding Sites” in GeneHancer (GH) sections with GH score greater than 1 and genes in “Interacting Proteins for FOXO3 Gene” sections. We also analyzed the peak count data of selected TFs from a database with uniformly processed ChIP-seq data named GTRD ( http://gtrd.biouml.org/ ) to demonstrate the candidate binding sites in Supplementary Fig. 10a . Bulk RNA-seq library preparation and sequencing After quantification of the RNA obtained from various cell types derived from hESCs [7] , [33] , [63] , sequencing libraries were generated using NEBNext ® Ultra™ RNA Library Prep Kit for Illumina ® (NEB) according to the manufacturer’s recommendations. At last, the library preparations were sequenced on an Illumina Hiseq X platform and 125 bp/150 bp paired-end reads were generated. Bulk RNA-seq analysis Quality control was performed by removing short reads (length < 37 bp) or low-quality reads ( N > 10%). After quality control, clean reads were aligned to human genome hg19 (UCSC; http://genome.ucsc.edu/ ) [64] using TopHat [45] (version 2.0.12). Then uniquely aligned reads were counted by HTseq [46] and assembled with Cufflinks [65] to get FPKM. DEGs were identified by DEseq2 [66] . CNV analysis Raw data of whole-genome DNA sequencing were first quality controlled by removing short reads (length < 37 bp) or low-quality reads ( N > 10%), and then clean reads were mapped to the human genome hg19 (UCSC) [67] , [68] using the software Bowtie2 [69] . After mapping, reads were sorted, and PCR duplicates were removed using SAMtools [70] . Only uniquely aligned reads were used to calculate the CNV using the software readCounter and R package HMMcopy [71] (version 1.21.0) in each 1 Mb window. The CNV was plotted by R package “circlize” [72] . ATAC-seq library preparation and sequencing ATAC-seq library was constructed according to the manufactory’s instructions with minor modification [73] . In brief, a total of 30,000 cells were lysed in lysis buffer for 10 min on ice. Immediately after lysis, nuclei were spun at 500 g for 5 min to remove the supernatant, following by incubation in 50 μL transposition reaction mix of TruePrepTM DNA Library Prep Kit V2 for Illumina (Vazyme Biotech) at 37 o C for 30 min. After stopping the tagmentation, PCR was performed to amplify the library for ten cycles. Then the amplified libraries were purified with 1.2× AMPure (Beckman) beads. Finally, the ATAC library was sequenced on an Illumina Hiseq X platform according to the manufacturer’s recommendation. ATAC-seq analysis First, raw data of ATAC-seq was quality controlled and mapped to hg19 (UCSC) [67] , [68] by Bowtie2 [69] as the same pipeline of the CNV analysis shown above. And then, mapped reads were sorted, PCR duplicates and reads from mitochondria were removed, and multiple aligned reads ( q < 30) were filtered out by SAMtools [70] . deepTools [74] was applied to check if the correlation between the replicates of each cell line is high. Then, bam files were transferred to bed files and called peaks by software MACS2 [75] . The identified peak regions were used to find enriched TF motifs by fndMotifsGenome.pl of the software Homer [76] . After calling peaks, the reproducible peaks between the replicates were identified by the software irreproducible discovery rate, and merged into a master peak list by function merge in bedtools [77] . The number of clean and uniquely mapped reads were counted by function intersect of bedtools [77] . The count matrix of all cell lines we collected was normalized into count per million (CPM). The Log scaled CPM was used to calculate the Pearson correlation coefficients among all samples. Western blotting Monkey tissues were homogenized in liquid nitrogen, lysed in 1% SDS buffer and further treated with a mechanical homogenizer. Cultured cells were lysed in 2× SDS and boiled at 105 °C for 10 min. Proteins (20 μg/lane) were electrophoresed on an SDS-PAGE gel and electrotransferred to polyvinylidene fluoride membranes (Millipore). Antibodies used in the present study are included in Supplementary Data 5 . Quantitative PCR (qPCR) Total RNA was extracted with TRIzol reagent (Invitrogen) according to the manufacturer’s instructions. For cDNA synthesis, 2 μg of total RNA was reverse transcribed into cDNA with Reverse Transcription Master Mix (Promega). qPCR reactions were performed in 384-well plates on a CFX-384 thermocycler (Bio-Rad) using iTaq Universal SYBR Green Supermix (Bio-Rad) according to the manufacturer’s instructions. Primer sequences for the experiment are listed in Supplementary Data 3 . ChIP-qPCR Cells were cross-linked using formaldehyde and lysed with SDS lysis buffer [78] . Subsequently, chromatin from the cells was sheared using a Covaris S2 instrument. After centrifugation, the supernatants were incubated overnight with Protein A Dynabeads bound to 2.4 μg of anti-FOXO3A, FOXA2 antibody, or rabbit IgG (sc-2027, Santa Cruz). After elution at 68 °C for 2 h, DNA was purified by phenolchloroform-isoamylalcohol and chloroform-isoamylalcohol extractions. The enriched DNA was subjected to qPCR to evaluate target protein occupation at the GLUL or FOXO3A promoter region. The primer sequences used for ChIP-qPCR are listed in Supplementary Data 3 . Histology and immunofluorescence staining For histological analysis, vessels were harvested, fixed with paraformaldehyde and stained with hematoxylin and eosin [7] . Frozen sections of vessels or cultured cells were fixed with ice-cold acetone and then subjected to immunofluorescence staining using an established protocol [79] . TrueVIEW Autofluorescence Quenching Kit (Vector, SP-8400) was used to reduce tissue autofluorescence. Detailed information about the antibodies is listed in Supplementary Data 5 . Calcium and lipid deposition was evaluated by von Kossa and Oil red O staining, respectively, as previously described [44] . Collagen fibers were histochemically detected by Sirius Red staining (Abcam, ab150681). Alexa Fluor™ 488 Ac-LDL (Invitrogen, L23380) was used to monitor the uptake ability of ECs. Images were visualized and captured using a Vectra Automated Quantitative Pathology Imaging System (Perkin Elmer), an Olympus DP72 microscope or a Leica SP5 confocal microscope. Quantitative analyses were performed on more than three slices, with three images per slice and >200 randomly selected cells per image if applicable, from each monkey using ImageJ software. Cell culture Wild-type hESCs (Line H9, Wicell) and derived FOXO3A −/− hESCs were cultured on Mitomycin C-inactivated mouse embryonic fibroblasts with cDF12 medium or Matrigel-coated plates with mTeSR1. HAECs and HUVECs were purchased from Lonza (Catalog # 2535 and C2519A). heVECs, HAECs, and HUVECs were maintained on collagen-coated plates in EGM2 medium supplemented with 10 nM SB431542, 50 ng/mL VEGF and 20 ng/mL bFGF. heVSMCs were cultured in VSMC medium with 10 ng/mL PDGF-AB. Human ESCs derived-MSCs were obtained and cultured in α-MEM medium supplemented with 10% fetal bovine serum, 0.1 mM nonessential amino acids, 1% penicillin/streptomycin, and 1 ng/mL bFGF. Human ESC-derived NSCs were obtained and cultured in NSC culture medium containing 50% Advanced DMEM/F12, 50% Neurobasal, 1× N2, 1× B27, 2 mM GlutaMAX, 10 ng/mL of human leukemia inhibitory factor (hLIF), 3 μM CHIR99021 and 2 μM SB431542. No mycoplasma contamination was observed during cell culture. Generation of FOXO3A -knockout hESCs Targeted gene knockout was fulfilled by TALEN-based homologous recombination [63] . Briefly, TALEN vectors (TAL2268, Plasmid #36705; TAL2269, Plasmid #36706) were purchased from Addgene. The 1.1-kb and 1.3-kb homology arms were amplified from the genomic DNA of hESCs and cloned into a donor plasmid. Primers used in the construction are included in Supplementary Data 3 . Both donor and TALEN vectors were electroporated into H9 hESCs. After ~2 weeks of selection, G418-resistant ESC clones were selected and expanded for further characterization. Karyotyping analysis A standard G-banding analysis was performed on the FOXO3A-knockout hESCs following the standard protocol [44] . Directed differentiation of hESCs into heVECs Briefly, after 1-day culture in mTeSR1 medium (STEMCELL Technologies), cells were transferred to M1 medium containing EC basal medium plus IWP2 (3 μM), CHIR99021 (3 μM), BMP4 (25 ng/mL), and basic fibroblast growth factor 2 (bFGF2) (4 ng/mL) for 3 days. M1 medium was replaced with M2 medium containing EC basal medium plus bFGF (20 ng/mL), vascular endothelial growth factor (VEGF) (50 ng/mL), and IL6 (10 ng/mL) for another 3 days to induce differentiation. Six days after induction of differentiation, adherent cells were harvested. Flow cytometry detection of the cell surface antigens (CD201 and CD34) and cell sorting were performed on a BD FACS Aria II. For heVECs transplantation assay, 1 × 10 6 heVECs were injected into four sites of the thigh muscles of the hindlimb ischemia mouse model. Blood perfusion was monitored every 4 days after the surgery by a laser Doppler blood perfusion (Moor instruments) [33] . Flow cytometry analysis For cell cycle analysis, 3 × 10 5 cells were fixed with 70% ethanol at −80 °C overnight and incubated in staining buffer containing 0.1% Triton X-100, 0.02 mg/mL propidium iodide and 0.2 mg/mL RNase A at 37 °C for 0.5 h, then analysis by FACS. For the measurement of NO, about 5 × 10 5 ECs were treated with DAF-FM (Molecular Probes, Invitrogen) for 30 min at room temperature. After staining, cells were analyzed by FACS. For Dil-Ac-LDL uptake assay, ECs were incubated with Dil-Ac-LDL for 6 h then analyzed by FACS. All experiments were performed on a BD LSRFortessa cell analyzer. RNA interference To knockdown FOXO3 or FOXA2 expression, we transfected corresponding siRNAs or nontarget siRNAs into ECs using Lipofectamine 3000 (Invitrogen). Briefly, 50 μM of FOXO3 or FOXA2 siRNA was mixed with 200 μL of Opti-MEM (Gibco) and 5 μL Lipofectamine 3000 and then added to one well of six-well plates. After a 6-h incubation, the culture medium was replaced with fresh medium. FOXO3 and FOXA2 siRNAs were synthesized by RIBOBIO, and siRNA sequences are listed in Supplementary Data 3 . Animal experiments Teratoma-forming assay was performed with 3 × 10 6 hESCs collected and injected into the legs of male NOD-SCID mice (6–8 weeks). After about two months, teratomas were analyzed by immunostaining. The hindlimb ischemia was performed in male BALB/c nude mice (8–10 weeks). In brief, the proximal and distal femoral artery were ligated using nonabsorbable suture (7–0) and 3 million ECs or PBS (negative control) were then injected into the ischemic hindlimb of the mice. Blood perfusion was monitored every four days by the laser Doppler blood perfusion (Moor instruments). SA-β-gal staining In brief, cells were fixed with fixation buffer (2% formaldehyde and 0.2% glutaraldehyde) for 3–5 min at room temperature. Then, cells were washed twice with PBS and stained with staining buffer at 37 °C overnight. The percentage of SA-β-gal positive cells were quantified using ImageJ. Clonal expansion assay Three thousand heVECs or heVSMCs were seeded in each collagen-coated well and cultured in complete heVEC and heVSMC medium for 10 days. Cells were fixed and stained with 0.2% crystal violet. The relative cell number was counted with ImageJ. Cell migration assay The cell migration ability of heVECs was measured by wound healing assays. For the wound healing assay, heVECs were plated and cultured in collagen-coated 12-well plates. When the cells reached 100% confluence, a linear scratch (“wound”) was generated using a 1-ml pipette tip, and the cells were cultured and monitored by IncuCyte live-cell analysis system (Essen BioScience) at 37 °C. The number of cells that migrated into the scratch was counted using ImageJ. In vitro Matrigel tube formation assay In brief, 7 × 10 4 ECs were seeded in Matrigel-coated 24 well plates. After 8 h of incubation, photographs were taken by the optical microscope (Olympus) and the tube length was quantified in three random microscopic fields with ImageJ. Luciferase reporter assay For luciferase reporter assay, FOXO3A promoter (−1980 to −992 bp) (containing the FOXA2 binding sites) were cloned into pGL3 vector. Then, HAECs were co-transfected with 0.8 μg of pGL3-FOXO3A-promoter vector, 0.2 μg of Renilla vector and 0.3 μg of FOXA2 cDNA expression vector (Origene, RC211408) or 50 uM siRNA-FOXA2. At 72 h after transfection, cells were lysed and relative luciferase activity was measured using Dual-Luciferase Reporter Assay Kit (Vigorous Biotechnology). Statistical analysis Data are presented as the means ± SEM. p value was calculated using GraphPad Prism software by two-tailed Student’s t tests. For multiple comparisons, two-way ANOVA or one-way ANOVA, followed by the recommended Holm–Sidak method, was used. Alternatively, statistical methods were included in figure legends. Ethics statement All animal experiments were conducted according to animal protocols approved by the Chinese Academy of Science Institutional Animal Care and Use Committee. Mice and monkeys were housed under a 12-h light/dark cycle and supplied with food and water ad libitum. Mice were anesthetized using isoflurane and euthanized with CO 2 followed by cervical dislocation. Reporting summary Further information on research design is available in the Nature Research Reporting Summary linked to this article.